Ancient origins determine global biogeography of hot and cold desert cyanobacteria Factors governing large-scale spatio-temporal distribution of microorganisms remain unresolved, yet are pivotal to understanding ecosystem value and function. Molecular genetic analyses have focused on the influence of niche and neutral processes in determining spatial patterns without considering the temporal scale. Here, we use temporal phylogenetic analysis calibrated using microfossil data for a globally sampled desert cyanobacterium, Chroococcidiopsis , to investigate spatio-temporal patterns in microbial biogeography and evolution. Multilocus phylogenetic associations were dependent on contemporary climate with no evidence for distance-related patterns. Massively parallel pyrosequencing of environmental samples confirmed that Chroococcidiopsis variants were specific to either hot or cold deserts. Temporally scaled phylogenetic analyses showed no evidence of recent inter-regional gene flow, indicating populations have not shared common ancestry since before the formation of modern continents. These results indicate that global distribution of desert cyanobacteria has not resulted from widespread contemporary dispersal but is an ancient evolutionary legacy. This highlights the importance of considering temporal scales in microbial biogeography. Microorganisms occur in all biomes and carry out essential biogeochemical functions and interactions with macroorganisms [1] . Understanding spatio-temporal patterns of microbial diversity and how they are determined is therefore relevant to all realms of ecology, with important implications for understanding ecosystem heterogeneity, conservation value and bioprospecting [2] . Although considerable effort has focused on the environmental drivers of community assembly [3] , relatively little is known about the factors that determine microbial biogeographic patterns for a given taxon, largely due to limitations of ineffective phylogenetic resolution and sampling of taxa and a lack of consideration of temporal scales [4] . Current dogma is supported by key phylogenetic studies on thermophilic prokaryotes, in which a positive correlation between geographic distance and genetic distance for populations has been shown [5] , [6] . Such studies have addressed spatial variability without considering the temporal scale, and we hypothesized that doing so would yield additional and critical insight on this issue. Deserts provide ideal model systems for large-scale microbial biogeographic studies, as they comprise the most abundant terrestrial biome on the Earth [7] and are relatively low energy systems that share readily identifiable major environmental stressors (that is, water availability and temperature [8] ) and a relative lack of confounding effects from grazing organisms. Deserts may also be likened to islands, as they are not spatially contiguous. The proximity of hot and cold deserts within the same continental regions provides natural controls to test hypotheses related to global distribution patterns, specifically, the extent that distribution of microorganisms reflects allopatric or selective forces. Here, we present a comprehensive analysis using a globally derived data set of the hypolithic cyanobacterial genus Chroococcidiopsis , which are common primary producers occurring in both hot [9] , [10] and cold [11] , [12] extreme arid deserts. A temporally scaled phylogenetic analysis combined with massively parallel pyrosequencing of environmental samples revealed distribution was dependent on contemporary climate and Chroococcidiopsis variants were specific to either hot or cold deserts. Within each climatically defined group, strong endemic signals were also recorded. Temporal phylogenies showed no evidence of recent inter-regional gene flow and indicated populations have not shared common ancestry since before the formation of modern continents. No evidence for distance-related patterns was detected. This study emphasizes the value of considering temporal scales in addition to spatial and environmental factors in microbial biogeography. Global sampling of desert environments We assembled an extensive sequence-based data set for the ubiquitously distributed desert cyanobacterial genus Chroococcidiopsis from every major desert on the Earth ( Fig. 1 ). These habitats included both hot and cold desert climates. We successfully recovered environmental DNA from hypolithic cyanobacterial biomass on translucent quartz. Clone libraries generated from each environmental sample were screened for Chroococcidiopsis phylotypes by analysis of 16S rRNA gene sequences and their 16S rRNA, 5.8S ITS and 23S rRNA loci were then sequenced for phylogenetic analysis. A total of 73 unique phylotypes were identified and sequenced ( Supplementary Table S1 ). 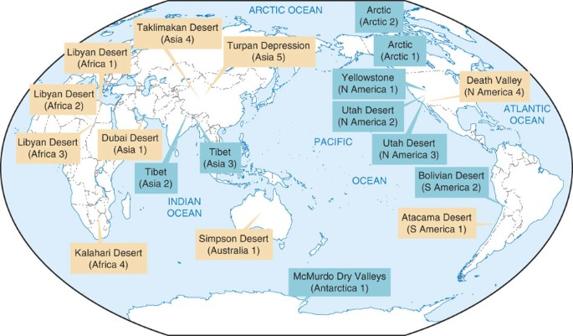Figure 1: Global distribution ofChroococcidiopsisvariants. The map indicates hot (brown boxes) and cold (blue boxes) desert locations from which variants were recovered. Detailed site descriptions and climatic information are given inSupplementary Table S1. Figure 1: Global distribution of Chroococcidiopsis variants. The map indicates hot (brown boxes) and cold (blue boxes) desert locations from which variants were recovered. Detailed site descriptions and climatic information are given in Supplementary Table S1 . Full size image Hypothetical scenarios for microbial biogeography This globally derived data set allowed for the testing of specific ecological and evolutionary scenarios ( Fig. 2 ). If microbial dispersal were ubiquitous without environmental selection, random patterns of distribution would emerge ( Fig. 2a ). These deserts would effectively present a single-microbial habitat and biogeographic province [3] . Alternatively, if geographic isolation, rather than environmental selection, were the main driver of diversity then location-specific lineages would arise in different provinces regardless of microhabitat ( Fig. 2b ). For example, hot and cold deserts in the North America would share common ancestry. Finally, in a scenario in which environmental selection drives diversification lineages consisting of bacteria from cold and hot habitats would be observed ( Fig. 2c ). For example, the cyanobacteria from hot desert in Death Valley would share ancestry with hot deserts from other continents rather than with cyanobacteria from cold desert in Utah. 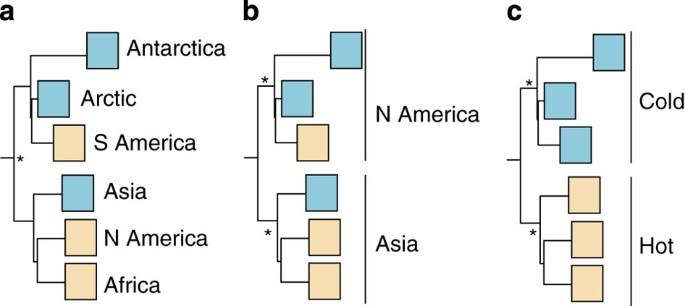Figure 2: Idealized phylogenies of hypothetical scenarios for global distribution of desert cyanobacteria. Scenarioa, assumes ubiquitous distribution resulting in mixed geographic regions and mixed environments within a phylogeny. Here, root divergence is a relatively recent event. Scenariob, assumes allopatric speciation resulting in distinct geographic regions and mixed environments within a phylogeny (that is, N America and Asia are monophyletic groups). Here, root divergence times correspond with formation of continents. Scenarioc, assumes environmental selection corresponding to global climatic change, resulting in a phylogeny with mixed geographic regions and distinct environments. Here, the root divergence times are significantly older than known ages of formation of continents. Asterisks indicate monophyletic groups. Brown boxes and blue boxes indicate hot and cold desert locations, respectively. Figure 2: Idealized phylogenies of hypothetical scenarios for global distribution of desert cyanobacteria. Scenario a , assumes ubiquitous distribution resulting in mixed geographic regions and mixed environments within a phylogeny. Here, root divergence is a relatively recent event. Scenario b , assumes allopatric speciation resulting in distinct geographic regions and mixed environments within a phylogeny (that is, N America and Asia are monophyletic groups). Here, root divergence times correspond with formation of continents. Scenario c , assumes environmental selection corresponding to global climatic change, resulting in a phylogeny with mixed geographic regions and distinct environments. Here, the root divergence times are significantly older than known ages of formation of continents. Asterisks indicate monophyletic groups. Brown boxes and blue boxes indicate hot and cold desert locations, respectively. Full size image Ancient times of common ancestry for extant Chroococcidiopsis A temporal phylogeny calibrated using fossil records [13] , [14] that have been shown as robust calibration points for cyanobacterial phylogenies [15] , was constructed using a Bayesian relaxed-clock analysis of the complete, unambiguously aligned, 16S-ITS-23S rRNA gene regions to estimate the divergence times of the globally distributed Chroococcidiopsis variants ( Fig. 3 , Supplementary Figs S1–S5 show all individual and combined gene trees). We used a relaxed phylogenetic approach [16] to estimate phylogeny and divergence times while taking into account uncertainties in evolutionary rates and calibration times [17] . Briefly, a 16S rRNA gene cyanobacterial phylogeny was constructed using the age of two fossilized ancestors as calibration points for estimation of evolutionary rates and timing of divergence events ( Supplementary Fig. S1 ). The estimated age of the common ancestor for Chroococcidiopsis was then incorporated as a previous constraint on subsequent Bayesian relaxed-clock analysis of the complete, unambiguously aligned, 16S-ITS-23S rRNA gene regions to estimate the divergence times of the globally distributed Chroococcidiopsis variants ( Supplementary Figs S2–S5 ). 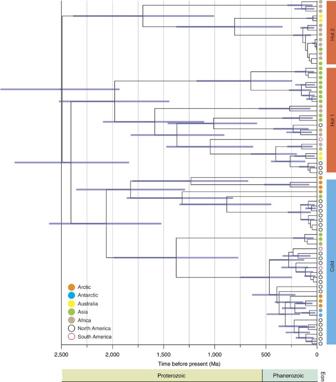Figure 3: Temporal phylogeny forChroococcidiopsisvariants. Variants were recovered from hot and cold deserts worldwide as shown inSupplementary Table S1. The tree was generated using a Bayesian relaxed-clock phylogenetic approach16of the 16S-ITS-23S rDNA regions to estimate divergence dates. The age of the common ancestor forChroococcidiopsiswas estimated with a 95% Bayesian confidence interval, using fossil ancestors for calibration13,14. Blue bars at nodes indicate 95% credible intervals for divergence events. Temporal scale is shown in millions of years. Figure 3: Temporal phylogeny for Chroococcidiopsis variants. Variants were recovered from hot and cold deserts worldwide as shown in Supplementary Table S1 . The tree was generated using a Bayesian relaxed-clock phylogenetic approach [16] of the 16S-ITS-23S rDNA regions to estimate divergence dates. The age of the common ancestor for Chroococcidiopsis was estimated with a 95% Bayesian confidence interval, using fossil ancestors for calibration [13] , [14] . Blue bars at nodes indicate 95% credible intervals for divergence events. Temporal scale is shown in millions of years. Full size image Our results showed hot and cold desert variants were evolutionarily distinct. All cold variants were monophyletic, whereas hot variants formed two groups with one sharing an ancient common ancestor with cold variants ∼ 2.4 Ga ( Fig. 3 , hot clade 1) and another ancestral to all extant Chroococcidiopsis variants ( ∼ 2.5 Ga; Fig. 3 , hot clade 2). The temporal phylogeny suggests that the time of most recent common ancestry to all contemporary variants was 2.5 Ga (range: 3.1–1.9 Ga) with a mean substitution rate estimate of 2.7×10 −5 substitutions/site/Ma (95% Bayesian confidence interval 2.0–3.5×10 −5 ; Fig. 3 , Supplementary Table S2 ). Within each clade, regionally distinct populations were apparent. For example, within the hot clade all variants from the Turpan Depression (Asia 5 in Supplementary Figs S1–S5 ) were monophyletic and share a common ancestor from ∼ 600 Ma. Region-specific lineages were apparent towards the tips of the phylogenetic trees, but the most recent times of common ancestry were ∼ 100 Ma ( Fig. 3 ). Evidence of gene flow between climatically similar deserts was also supported from the phylogenetic analysis. For example, within the last 100 million years a population of African variants from the Libyan Desert, Egypt (Africa 2) likely established a founder population in the Taklimakan Desert, China (Asia 4) and links African and Asian variants within the hot 2 clade ( Supplementary Fig. S2 ). But, in all cases, where such events could be detected these were ancient divergences and rare. Absence of invasive colonization between deserts We also carried out massively parallel rRNA gene directed metagenomic 454 pyrosequencing of hot and cold desert environmental samples, targeting the highly variable V5-V7 16S rRNA gene region to identify possible 'rare' phylotypes not recovered in our clone libraries [18] , [19] ( Supplementary Table S3 ). This analysis showed that contemporary hot and cold clade Chroococcidiopsis variants were exclusive to hot and cold deserts, respectively, with the exception of a single cold clade variant that was recovered from the hot desert at very low abundance (<0.05%) within the assemblage. Hot variants did, however, share greatest phylogenetic affiliation with variants from their own rather than any other climatically similar desert. Therefore, dispersal and establishment of hot variants in cold deserts ( P =0), and vice versa ( P =0.002), were extremely rare events. Distance–decay patterns do not explain global scale distribution Effects of climatic and substrate variables were evaluated by analysis of molecular variance (AMOVA, incorporating F Statistic) and phylogenetic test (P-test), whereas the effects of distance-related variables were assessed using the Mantel Statistic. Contemporary climate classification based on long-term mean annual temperature and precipitation data was significant in differentiating hot and cold clades (AMOVA, F CT =0.29147, P <0.00001). The phylogenetically informed delineation into 'hot' and 'cold' groupings provided the most parsimonious explanation (P-test, P <0.001) for the observed tree topology. On a global scale, genetic differentiation was not related to geographic distance (Mantel, R 2 =0.0055, P =0.169; Fig. 4a ) or altitude (Mantel, R 2 =0.0011, P =0.601) for the homogenous substrate either within or between these major clades. We further tested the genetic and geographic distance relationship of the phylogenetically identified cold, hot 1 and hot 2 clades by the same method. On this more refined genetic scale, we were also unable to infer a correlation between genetic divergence and geographic distance ( Fig. 4b–d ). Analysis of relatively close desert locations showed a lack of relatedness between variants from the hot Death Valley desert versus the cold Utah Desert in North America (AMOVA, F ST =0.84053, P =0.00586), the warm Turpan Depression versus the cold Tibetan tundra in China (AMOVA, F ST =0.74756, P =0.00391), and the warm Atacama Desert versus the cold high altitude Bolivian Desert in South America (AMOVA, F ST =0.93831, P <0.00001), whereas Antarctic variants were most closely affiliated with Arctic variants (F ST =0.35368, P =0.18359). 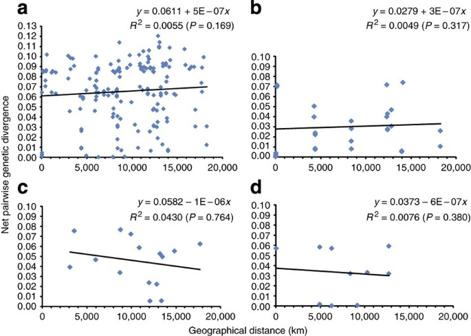Figure 4: Relationship between genetic divergence and geographic distance amongChroococcidiopsisvariants. Genetic differentiation was not significantly related to geographic distance (a) on the global scale (N=19,n=171), or for each of the phylogenetically defined clusters (b) cold (N=8,n=28), (c) hot 1 (N=6,n=15) or (d) hot 2 (N=5,n=10); whereNdenotes number of samples andnthe resultant number of pairwise comparisons. The best-fit linear regression function, the coefficient of determination (R-square) and significance (p) of Mantel test are displayed for individual regression plots. A significance level (alpha) of 0.05 was applied. Figure 4: Relationship between genetic divergence and geographic distance among Chroococcidiopsis variants. Genetic differentiation was not significantly related to geographic distance ( a ) on the global scale ( N =19, n =171), or for each of the phylogenetically defined clusters ( b ) cold ( N =8, n =28), ( c ) hot 1 ( N =6, n =15) or ( d ) hot 2 ( N =5, n =10); where N denotes number of samples and n the resultant number of pairwise comparisons. The best-fit linear regression function, the coefficient of determination (R-square) and significance ( p ) of Mantel test are displayed for individual regression plots. A significance level (alpha) of 0.05 was applied. Full size image The temporal phylogeny generated divergence time estimates that broadly concur with estimates for the onset of widespread aridity on the Earth ( ∼ 1.8 Ga) [8] . Interestingly, the estimated substitution rate was approximately an order of magnitude lower than estimates for other bacterial groups [20] . This further supports the suggestion that a universal evolutionary rate may not exist for all bacteria [20] . The majority of divergences within the temporal phylogeny that explain diversity of extant Chroococcidiopsis variants were ancient and pre-date the estimated onset of contemporary aridity for many locations. For example the oldest contemporary arid region is thought to be the Namib Desert ( ∼ 80 Ma [21] ). The North African, the Polar, the South American and the Tibetan aridity have likely persisted since 30–45 Ma [22] , [23] , [24] , [25] , [26] , [27] , whereas others such as the Death Valley, the Simpson and the Taklimakan deserts may be relatively recent [28] , [29] , [30] . Despite regionally specific monophyletic clades within both hot and cold clades, the times of common ancestry for Chroococcidiopsis variants pre-dated estimates for contemporary aridity in these desert regions. This suggests that the global distribution for Chroococcidiopsis has been limited by barriers to long distance dispersal and/or invasive colonization, with regional gene pools maintained over geological timescales. Environmental selection may also have exerted a major role in colony establishment in different geographical regions. Similar to our results, DNA fingerprinting studies of Pseudomonas isolates from soil showed that strains were not globally mixed, but rather regionally endemic strains had evolved [31] . The high-coverage sequencing of environmental samples further indicated that the hot and cold delineation for Chroococcidiopsis variants is valid ecologically, as variants were exclusive to either hot or cold deserts. From our data it is reasonably concluded that dispersal and establishment of hot variants in cold deserts, and vice versa, are extremely rare events. As phylotypes were more similar to those from their own rather than any other climatically similar desert, this also suggests a lack of dispersal between similar habitats. The temporal phylogeny therefore strongly indicates that variants within hot and cold clades do not readily disperse and colonize climatically similar deserts. Although founder populations may establish colonies in other climatically similar regions, our data suggests these events were rare. Whereas it is possible that a population of African variants from the Libyan Desert, Egypt, established a founder population in the Taklimakan Desert, China, within the last 100 million years, linking both African and Asian variants within the hot 2 clade, similar events were apparently rare despite the very long evolutionary timescales. Additional examples were evident in the phylogenetic trees, but it was unlikely that any establishment of new populations in these geographically distant locales was a recent event. This further indicates that dispersal events between these desert locations could be limiting and/or invasive colonization rarely succeeds. Our phylogeny thus becomes predictive for evolutionary lineage in a given climatically defined desert. The different populations recovered from locations in relatively close proximity, but experiencing different climates illustrated how differentiation of Chroococcidiopsis variants can be explained by adaptation to climate-driven selection pressures on the bacterial population rather than distance between populations. For example, the lack of relatedness between variants from the hot Death Valley desert versus the cold Utah Desert in North America, the warm Turpan Depression versus the cold Tibetan desert in China or the warm Atacama Desert versus the cold high altitude Bolivian Desert in South America. This contrasted with highly similar populations from Antarctic and Arctic locations, strongly suggesting geographic distance has little affect on divergence or relatedness between populations. We also demonstrated that distance-related patterns were not apparent on a global scale for variants adapted to similar environments (that is, within hot or cold clades), suggesting that distance–decay relationships may not be applicable to this globally distributed bacterium. This is in contrast to the notion of distance–decay relationships between genetic and geographic distance among microbial populations [2] , [3] , [4] , [5] , [6] . Recent experimental studies have demonstrated that at the community level, distance–decay patterns may be observed in the short term (<7 days) but have a relatively minor role over longer time periods [32] . Although an increased interest in microbial biogeography has lead to a re-examination of the distance–decay explanation of bacterial distribution patterns for various communities [2] , [3] , [4] , there nonetheless remains insufficient data to reject this hypothesis or support alternatives to describe microbial distribution, community structure or genetic variation. We hypothesize that acquisition of adaptive traits facilitating speciation into cold desert variants was an ancient event that evolved in globally dispersed ancestral hot-adapted Chroococcidiopsis variants. The ancestral variant is a likely candidate for early terrestrial life during the Earth's long arid history [8] , [33] . We demonstrated that although a desert cyanobacterium such as Chroococcidiopsis may notionally possess the characteristics for ubiquitous dispersal due to aeolian transport of desert particulates and its desiccation/radiation tolerance [34] , [35] , this is not reflected in contemporary colonization patterns. The existence of regionally isolated gene pools of hot and cold Chroococcidiopsis variants strongly supports the concept that widespread contemporary dispersal is not common, and that relationships reflect ancient historical legacies [36] . Although strong selection for hot and cold variants has occurred, this pre-dates contemporary climatic selective pressures and so indicates that the complex interaction of allopatric and selective forces can be more fully understood by considering temporal scales in microbial biogeography. This also highlights a value for local microbial diversity and suggests that microorganisms are likely to face threats of reduced biodiversity due to local extinction in a manner similar to macroorganisms. Temporally calibrated phylogenetic data sets such as these may in future also help to inform issues in the reconstruction of ancient geomorphology and climate, in a manner analogous to records of colonization by macroorganisms [37] . Environmental samples We targeted the hypolithic niche (cyanobacterial colonization on the ventral surface of translucent quartz rock), as this inert and relatively homogeneous substrate is ubiquitous in desert pavement terrain. Hypoliths are photoautotrophs and so localized substrate-related effects on communities are minimized. Hypolithic communities dominated by cyanobacteria are clearly distinct from the surrounding soil biota [12] and long lived [10] . The combination of stable environment and a long-lived community reduces potential for bias due to short-term temporal variability. The cyanobacterial genus Chroococcidiopsis has monophyletic rRNA gene defined origins [38] and cyanobacteria have a documented micro-fossil [13] , [14] record that allows temporal phylogenies to be calibrated. We collected colonized white quartz rocks (hypoliths, N =54) from desert pavement terrain in desert locations worldwide ( Fig. 1 , Supplementary Table S1 ). Geographical distance between sites was calculated using the law of haversines. At least three hypoliths were collected from each location. Biomass was recovered aseptically and environmental DNA purified by phenol–chloroform extraction and ethanol precipitation. For each location we recorded precise location and this was mapped via geographic information system to a global climate map based on long-term mean annual temperature and rainfall [7] , [8] . The quartz (SiO 2 ) substrate was characterized using standard USGS mineralogical diagnostic criteria ( http://www.usgs.gov ). Recovery of Chroococcidiopsis variants Clone libraries (colonies/library, N ⩽ 50; total N = ⩽ 950) were generated from hypolith samples from each location using cyanobacteria-specific primers (359F-2763R) [39] , [40] spanning a contiguous region of loci with incremental rates of evolution including 16S rDNA, ITS and 23S rDNA. Libraries were screened for Chroococcidiopsis variants by sequencing (359F-781R) [40] (BigDye Terminator 3.1, 3730 Genetic Analyzer, Applied Biosystems). Individual phylotypes were identified from the environmental sample clone libraries by phylogenetic analysis of 16S rRNA gene sequences ( ∼ 550 bp) using distance criteria optimized with the Generalized Time Reversible model (GTR+I+G) (PAUP v4.0 (ref. 41 )). All unique clones that affiliated phylogenetically with Chroococcidiopsis were then sequenced along with the entire 16S rRNA, 5.8S ITS and 23S rRNA gene region comprising ∼ 4,300 bp ( Supplementary Table S4 ). Ambiguously aligned regions were excluded from all analyses. The final alignment was 3,645 bp ( N =73). Model selection was achieved using ModelTest [42] using the Akaike Information Criterion to choose the best-fit model. In all cases, the best-fit model was the GTR+I+G model and this was applied to each analysis. Relaxed-clock phylogenetic analyses Temporal phylogenies were generated using a Bayesian 'relaxed molecular clock' approach with a Bayesian skyride coalescent prior [16] , [43] . This prior does not require strong a priori decisions about the demographic history of the population (that is, number of coalescent events) and was used in all analyses. Initially, 16S rRNA genes of a broad cross-section of cyanobacterial orders, including Chroococcales, Nostocales, Oscillatoriales, Pleurocapsales, Prochlorales, Stigonematales and plastids available from the NCBI GenBank were used ( N =224, Supplementary Fig. S1 ). Two fossilized ancestors for the cyanobacterial families were used as calibration points for estimation of evolutionary rates and timing of divergence events [13] , [14] . Tests for congruence between the complete data set ( Supplementary Fig. S2 ) and among trees generated from different loci ( Supplementary Figs S3–S5 ) were made using the Shimodaira–Hasegawa test [44] ( Supplementary Table S5 ). The estimated age of the common ancestor for Chroococcidiopsis was then incorporated as a previous constraint on subsequent Bayesian relaxed-clock analysis of the complete, unambiguously aligned, 16S-ITS-23S rRNA gene regions ( ∼ 3.6 kbp) to estimate the divergence times of the globally distributed Chroococcidiopsis variants ( Supplementary Fig. S2 ). Massively parallel rRNA gene-directed pyrosequencing Environmental DNA from representative hot (Turpan Depression) and cold (central Tibet) desert hypoliths within the same continental region were selected for massively parallel pyrosequencing. Amplicons of the hyper-variable V5–V7 region of the 16S rRNA gene [18] were pyrosequenced using the Roche 454 Life Sciences GS-FLX sequencer (Taxon Biosciences). Pyrosequencing flowgrams were filtered and de-noised using a variation of the AmpliconNoise suite designed for FLX Titanium sequences. In short, reads with at least one flow of signal intensity between 0.5 and 0.7 or a cycle of four nucleotide flows (ATGC) that failed to give a signal >0.5 (both signs of noise) before flow no. 400 were discarded, and all reads were truncated at flow no. 600. Pyrosequencing noise was removed from filtered flowgrams using the PyroNoise [19] program with default settings, and PCR noise was removed from the resulting sequences using the SeqNoise [19] program ( σ s=0.033, cs=0.08) after they were truncated at 400 bp to further reduce noise. Last, the sequences were checked for PCR chimeras using Perseus (α=−7.5, β=0.5). The output sequences were annotated using Metagenome Rapid Annotation using Subsystem Technology to identify cyanobacteria-affiliated sequences [45] . Sequences that were 97% homologous to Chroococcidiopsis were further confirmed by DOTUR [46] and online BLAST tool ( Supplementary Table S3 ). Nucleotide sequence accession Nucleotide sequences generated in this study have been deposited to the NCBI GenBank database under accession numbers FJ805842 , FJ805957 (temporal phylogeny), HM453992 , HM454160 (cold desert pyrosequencing), HM489009 , HM489864 (hot desert pyrosequencing). Statistical analyses Effects of climatic and substrate variables were evaluated by AMOVA (incorporating F ST ) on nucleotide sequences and P-test [47] on tree topologies, whereas the effects of distance related variables (location, altitude) were assessed using the Mantel Statistic (Arlequin v3.1 (ref. 48 )) with significance testing against 1,000 permutations. Net genetic divergences were calculated using MEGA v4.1 (ref. 49 ). Normality was ensured before the computation of power functions using Linear Least Squares Fit regression analysis. Accession codes. Nucleotide sequences have been deposited in Genbank under accession codes FJ805842-FJ805957, HM453992-HM454160 and HM489009-HM489864. How to cite this article: Bahl, J. et al . Ancient origins determine global biogeography of hot and cold desert cyanobacteria. Nat. Commun. 2:163 doi: 10.1038/ncomms1167 (2011).